FOXO1 inhibition yields functional insulin-producing cells in human gut organoid cultures Generation of surrogate sources of insulin-producing β-cells remains a goal of diabetes therapy. While most efforts have been directed at differentiating embryonic or induced pluripotent stem (iPS) cells into β-like-cells through endodermal progenitors, we have shown that gut endocrine progenitor cells of mice can be differentiated into glucose-responsive, insulin-producing cells by ablation of transcription factor Foxo1. Here we show that FOXO1 is present in human gut endocrine progenitor and serotonin-producing cells. Using gut organoids derived from human iPS cells, we show that FOXO1 inhibition using a dominant-negative mutant or lentivirus-encoded small hairpin RNA promotes generation of insulin-positive cells that express all markers of mature pancreatic β-cells, release C-peptide in response to secretagogues and survive in vivo following transplantation into mice. The findings raise the possibility of using gut-targeted FOXO1 inhibition or gut organoids as a source of insulin-producing cells to treat human diabetes. Since 1922, lifelong insulin replacement has been the mainstay of type 1 diabetes treatment. Efforts to generate surrogate insulin-producing cells that could serve as a ‘permanent cure’ of the disease have been underway for nearly two decades, and progress has been made towards the generation of pancreatic hormone-producing cells from either embryonic stem or induced pluripotent stem cells (iPS) [1] , [2] , [3] . However, cells thus generated are often polyhormonal, and are characterized by an indifferent response to glucose, unless transplanted into mice, where they acquire undetermined factors required for their functional ‘maturation’ [2] , [4] . Although terminally differentiated β-cells are only present in the pancreas, endocrine progenitors with similar features to pancreatic endocrine progenitors are also found in the intestine, the site of the body’s largest endocrine system [5] . The enteroendocrine system is comprised of many different cell types, some of which are shared in common with the endocrine pancreas (for example, somatostatin- and ghrelin-producing cells), and some of which are organ-specific [5] . We have shown in previous work that genetic inactivation of Foxo1 (we use lower case for mouse and upper case for human gene products; italics for genes) in mice results in the expansion of the enteroendocrine Neurogenin3 (Neurog3)-positive progenitor cell pool, and the appearance of functional insulin-producing cells that express all markers of mature pancreatic β-cells, secrete insulin in response to physiologic and pharmacologic cues, and can readily regenerate to alleviate diabetes caused by the β-cell toxin streptozotocin [6] . These data did not arise in a vacuum; rather, they are part of a burgeoning body of evidence indicating that enteric and pancreatic endocrine cells can convert into different subtypes [7] , possibly through a dedifferentiation process [8] , [9] , [10] . In contrast to the mouse, little is known about the effect of FOXO1 on endocrine differentiation in the human gut, especially whether FOXO1 loss-of-function can alter the fate of enteroendocrine cells towards the insulin-producing lineage [11] . The present study was undertaken to assess the human relevance of the observation that deleting Foxo1 can promote the insulin-producing fate in experimental animals [6] , as a necessary preliminary step towards the therapeutic application of these observations to diabetic patients. We report here that FOXO1 expression defines endocrine progenitor and serotonin-positive cells in the human gut. Using gut organoid differentiation [12] of human iPS cells, we show that FOXO1 inhibition in FOXO1-expressing cells results in their conversion into insulin-positive cells that express markers of mature pancreatic β-cells. Further, we show that these cells secrete C-peptide in response to glucose, arginine and KCl. These data provide the required proof-of-principle to attempt to engineer insulin-producing cells from human gut organoid cultures, or to pursue direct FOXO1 inhibition in the human gut as approaches to type 1 diabetes treatment. Survey of FOXO1 localization in the human gut We used fluorescence immunohistochemistry to survey FOXO1 localization in the human gut ( Fig. 1 ). FOXO1-expressing cells were most abundant near the bottom of the crypts; 60% of FOXO1-positive cells were located between positions 0 to +9 relative to the crypt bottom in the duodenum and colon, with lower frequencies at positions more distal than +10, and in the jejunum and ileum ( Fig. 2a–d ). FOXO1 messenger RNA (mRNA) levels correlated with the abundance of FOXO1-immunoreactive cells ( Fig. 2e ). Intestinal lineage marker analysis indicated that FOXO1 expression was virtually restricted to CHROMOGRANIN A (CGA)-positive endocrine cells ( Fig. 1a–d ). FOXO1-positive cells (95.3±1.8%) were CGA positive, whereas 61.8±3.8% of CGA-positive cells had immunoreactivity with FOXO1 in three human duodenal specimens. FOXO1-positive crypt cells were OLFACTOMEDIN-4 (OLFM4)-negative ( Fig. 1e ), indicating that they are unlikely to be intestinal stem cells [13] . They were, however, immunoreactive with EPHB3, a pro-endocrine marker in pancreas [14] that localizes to columnar cells at the crypt base and Paneth cells ( Fig. 1c ) [15] . These findings are consistent with FOXO1-positive crypt cells being endocrine progenitors. But attempts to characterize these cells with NEUROG3 antibodies—a marker of pancreatic [16] , [17] and intestinal [18] endocrine progenitors—failed. We found that >80% of FOXO1-positive cells in villi were immunoreactive with serotonin antibodies and 85±11% of serotonin (5HT)-positive cells were FOXO1-positive ( Fig. 1h ). Interestingly, pancreatic β-cells also make serotonin [19] . In addition, FOXO1-immunoreactive cells showed reactivity with prohormone convertases (PC) 1/3 and 2 (refs 20 , 21 ), as well as the ATP-dependent potassium channel SUR1, an important protein for glucose-dependent insulin secretion in β-cells [22] ( Fig. 2f–n ). These findings indicate that FOXO1-positive gut cells share features with pancreatic β-cells. 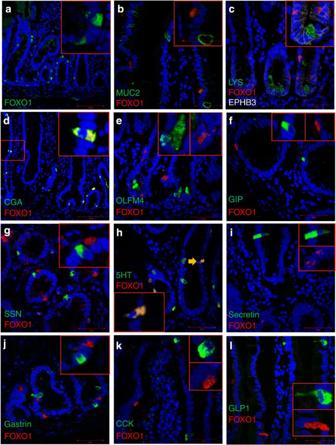Figure 1: Survey of FOXO1 expression in the human duodenum. (a–e) FOXO1 (red) colocalization with secretory markers, MUCIN2 (MUC2), LYSOXYME (LYS), CHROMOGRANINA (CGA), OLFACTOMEDIN-4 (OLFM4) (all green) and EPHB3 (grey). (f–l) Colocalization of FOXO1 with endocrine cell markers GIP, somatostatin (SSN), serotonin (5HT), secretin, gastrin, cholecystokinin (CCK) and GLP1. Scale bar, 100 μm ina–e, and 50 μm inf–l(n=3). Figure 1: Survey of FOXO1 expression in the human duodenum. ( a – e ) FOXO1 (red) colocalization with secretory markers, MUCIN2 (MUC2), LYSOXYME (LYS), CHROMOGRANINA (CGA), OLFACTOMEDIN-4 (OLFM4) (all green) and EPHB3 (grey). ( f – l ) Colocalization of FOXO1 with endocrine cell markers GIP, somatostatin (SSN), serotonin (5HT), secretin, gastrin, cholecystokinin (CCK) and GLP1. Scale bar, 100 μm in a – e , and 50 μm in f – l ( n =3). 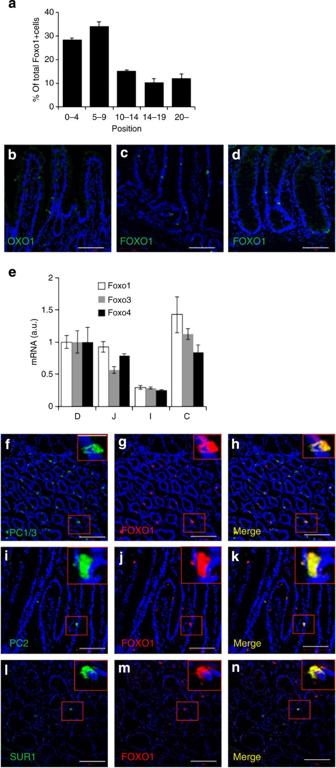Figure 2: Characterization of FOXO1-expressing cells in human gut. (a) Quantitative analysis of the position of FOXO1-positive cells in the human duodenum.(b–d) FOXO1 immunostaining in (b) jejunum, (c) ileum and (d) colon. (e) Quantitative PCR (qPCR) analysis ofFOXO1mRNA in human intestine (D, duodenum; J, jejunum; I, ileum; and C, colon). (f–n) Immunostaining of FOXO1 with PC1/3, PC2 and SUR1 in the human colon. Scale bar, 100 μm (n=3 for histology and qPCR) We present data as means±s.e.m. Full size image Figure 2: Characterization of FOXO1-expressing cells in human gut. ( a ) Quantitative analysis of the position of FOXO1-positive cells in the human duodenum. ( b – d ) FOXO1 immunostaining in ( b ) jejunum, ( c ) ileum and ( d ) colon. ( e ) Quantitative PCR (qPCR) analysis of FOXO1 mRNA in human intestine (D, duodenum; J, jejunum; I, ileum; and C, colon). ( f – n ) Immunostaining of FOXO1 with PC1/3, PC2 and SUR1 in the human colon. Scale bar, 100 μm ( n =3 for histology and qPCR) We present data as means±s.e.m. Full size image Generation and analysis of human gut organoids To assess the role of FOXO1 in human enteroendocrine cell differentiation, we generated gut organoids using three lines of human iPS cells derived from healthy donors [12] , [23] . Time course analyses with immunohistochemical markers indicated that CDX2-expressing cells appeared in 8-day-old organoids ( Fig. 3a ), followed by MUCIN (MUC2), LYSOZYME (LYS) and CGA-positive cells at day 14 of differentiation ( Fig. 3b–d ); we did not detect terminally differentiated enteroendocrine cells at this stage. 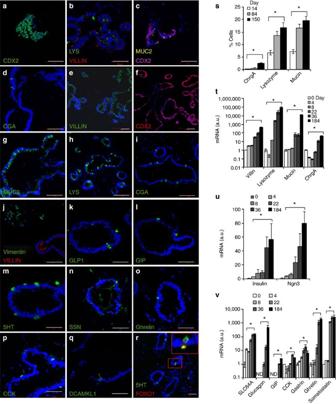Figure 3: Marker analysis of 150-day-old human iPS-derived gut organoids. (a) CDX2 (green) in 8-day-old organoids; (b) LYS (green) and VILLIN (red); (c) MUC2 (yellow) and CDX2 (magenta); (d) CGA (green) in 14-day-old organoids by immunohistochemistry. (e) Villin; (f) CDX2; (g) MUC2; (h) LYS; (i) CGA; (j) vimentin (green) and VILLIN (red) in 150-day-old gut organoids. (k–r) Analysis of endocrine cells; GLP1, GIP, 5HT, SSN, ghrelin, cholecystokinin (CCK), tuft cells (DCAMKL1), FOXO1 (green) and 5HT (red) in 150-day-old organoids. (s) Quantification of CGA-, LYS- and MUC2-positive cells by immunohistochemistry. (t–u) Time course quantitative PCR (qPCR) analysis ofVILLIN,LYSOZYME,MUCIN2andCGA(t);INSULINandNEUROG3(u);SLC6A4(serotonin transporter),GLUCAGON,GIP,CCK,GASTRIN,GHRELINandSSNduring gut differentiation. (v) Scale bar, 100 μm in panelsa–j; 50 μm in panelsk–r(n=3 each for histology and qPCR) (*P<0.05 by ANOVA). We present data as means±s.e.m. ND, not detected. Figure 3: Marker analysis of 150-day-old human iPS-derived gut organoids. ( a ) CDX2 (green) in 8-day-old organoids; ( b ) LYS (green) and VILLIN (red); ( c ) MUC2 (yellow) and CDX2 (magenta); ( d ) CGA (green) in 14-day-old organoids by immunohistochemistry. ( e ) Villin; ( f ) CDX2; ( g ) MUC2; ( h ) LYS; ( i ) CGA; ( j ) vimentin (green) and VILLIN (red) in 150-day-old gut organoids. ( k – r ) Analysis of endocrine cells; GLP1, GIP, 5HT, SSN, ghrelin, cholecystokinin (CCK), tuft cells (DCAMKL1), FOXO1 (green) and 5HT (red) in 150-day-old organoids. ( s ) Quantification of CGA-, LYS- and MUC2-positive cells by immunohistochemistry. ( t – u ) Time course quantitative PCR (qPCR) analysis of VILLIN , LYSOZYME , MUCIN2 and CGA ( t ); INSULIN and NEUROG3 ( u ); SLC6A4 (serotonin transporter), GLUCAGON , GIP , CCK , GASTRIN , GHRELIN and SSN during gut differentiation. ( v ) Scale bar, 100 μm in panels a – j ; 50 μm in panels k – r ( n =3 each for histology and qPCR) (* P <0.05 by ANOVA). We present data as means±s.e.m. ND, not detected. Full size image Gut organoids (150 days old) resembled human gut morphology, including mesenchymal and enteroendocrine cells ( Fig. 3e–r ). The secretory lineages marked by MUC2 and LYS were present at physiologic frequencies, while CGA-positive cells were twice as abundant in iPS-derived organoids as in the gut (2.6±0.2 vs 1.0±0.2%, P <0.05 by ANOVA) ( Fig. 3s ) [5] . Time course analyses of mRNA expression indicated that lineage markers increased exponentially during differentiation, with a notable step-up between day 8 and 22, coincidental with the transition from budding microspheres to tridimensional culture in matrigel ( Fig. 3t ). The presence and abundance of terminally differentiated enteroendocrine cells in human gut organoids has been characterized only in part [7] . We found that glucagon-like peptide 1 (GLP1)-, gastric inhibitory peptide-, somatostatin (SSN)-, cholecystokinin- and 5HT-positive cells first appeared in ~90-day-old organoids. In contrast, gastrin-, secretin-, substance P- and tufts cells appeared in 150-day-old organoids ( Fig. 3k–q ). Quantitative PCR analyses also revealed the time-dependent increases in mRNA levels of genes associated with endocrine progenitor and terminally differentiated enteroendocrine cells, including INSULIN ( Fig. 3u,v ; Supplementary Table 3 ). We compared the frequency of representative cell types (CGA, 5HT, GLP1 and SSN) in 230-day-old organoids with the human duodenum. We found that CGA- and GLP1-positive cells were approximately twice as abundant in organoids as in the duodenum; 5HT cells were present at comparable levels, whereas SSN cells were half as abundant in organoids compared with the duodenum ( Fig. 4a ). 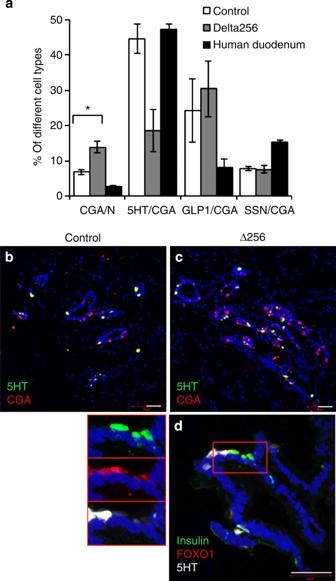Figure 4: Changes to enteroendocrine cells following FOXO1 inhibition. (a) Quantification of cells expressing CGA, 5HT, GLP1 and SSN in 230-day-old gut organoids transduced with control (empty bars), HA-Δ256 FOXO1 adenovirus (grey bars) or the human duodenum (black bars). (b–d) Immunohistochemistry with 5HT (green) and CGA (red) in 230-day-old gut organoids transduced with HA-Δ256 FOXO1 or control adenovirus. (d) Immunohistochemistry of insulin (green), FOXO1 (red) and 5HT (white) in 230-day-old gut organoids transduced with HA-Δ256 FOXO1 adenovirus. Insets on the left show magnifications of a cluster of 5HT-, FOXO1- and insulin-positive cells. Scale bar, 50 μm (n=3 for histology and quantitative PCR) (*P<0.05 vs organoids transduced with control shRNA lentivirus or HA-Δ256 adenovirus byt-test). We present data as means±s.e.m. Figure 4: Changes to enteroendocrine cells following FOXO1 inhibition. ( a ) Quantification of cells expressing CGA, 5HT, GLP1 and SSN in 230-day-old gut organoids transduced with control (empty bars), HA-Δ256 FOXO1 adenovirus (grey bars) or the human duodenum (black bars). ( b – d ) Immunohistochemistry with 5HT (green) and CGA (red) in 230-day-old gut organoids transduced with HA-Δ256 FOXO1 or control adenovirus. ( d ) Immunohistochemistry of insulin (green), FOXO1 (red) and 5HT (white) in 230-day-old gut organoids transduced with HA-Δ256 FOXO1 adenovirus. Insets on the left show magnifications of a cluster of 5HT-, FOXO1- and insulin-positive cells. Scale bar, 50 μm ( n =3 for histology and quantitative PCR) (* P <0.05 vs organoids transduced with control shRNA lentivirus or HA-Δ256 adenovirus by t -test). We present data as means±s.e.m. Full size image FOXO1 inhibition yields insulin-immunoreactive cells To determine whether human enteroendocrine cells can be manipulated to yield insulin-producing cells, we transduced 170-day-old organoids with adenovirus expressing a dominant-negative mutant FOXO1 (HA-Δ256) (ref. 24 ) and analysed them 2 weeks thereafter. mRNA analyses showed that gut organoids were efficiently transduced with this mutant, without affecting other FOXO isoforms ( Fig. 5a ). HA-Δ256 expression significantly increased transcripts of INSULIN , NEUROG3 , and CGA by eight-, six- and twofold, respectively ( Fig. 5b ) ( P <0.05 by t -test). It should be noted, however, that CGA transcripts were ~8,000-fold more abundant than NEUROG3 transcripts, and ~40,000-fold more abundant than INSULIN transcripts at this stage ( Supplementary Table 3 ). Immunohistochemical analyses of multiple differentiation experiments conducted with three separate iPS lines demonstrated the presence of insulin/C-peptide/CGA-positive cells ( Fig. 5c–f ). These cells represented 0.5% of CGA-positive cells in control organoids transduced with green fluorescent protein adenovirus (~2 of 5,000 cells scored in each experiment), but their frequency increased to ~5% in gut organoids expressing dominant-negative FOXO1 (~31 of 4,000 cells scored in each experiment) ( Fig. 5c ) ( P <0.05 by t -test). In the latter, immunohistochemistry demonstrated that insulin-positive cells were immunoreactive with HA antibodies, indicating that the induction of insulin immunoreactivity occurred in cells with inactivated FOXO1 ( Fig. 5g,h ). Not all hemagglutinin (HA)-positive cells were insulin-positive, possibly reflecting expression of the adenovirus in cells whose fate was not affected by FOXO1 ablation. Moreover, co-immunostaining with insulin and FOXO1 indicated that insulin-immunoreactive cells were invariably immunoreactive with cytoplasmic (that is, inactive) FOXO1 ( Fig. 5i,j ). Immunostaining with insulin and CDX2 or αSMA (a marker of mesenchymal cells) showed that insulin-positive cells were immunoreactive with the former, but not with the latter, making it unlikely that the insulin-positive cells result from epithelial–mesenchymal transition ( Fig. 5k,l ). 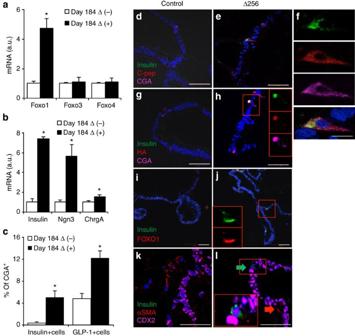Figure 5: Insulin-positive cells in 184-day-old human gut organoids. (a,b) Quantitative PCR (qPCR) analysis of different markers in gut organoids transduced with control (empty bars) or HA-Δ256 FOXO1 adenovirus (black bars). (c) Quantification of insulin- and GLP1-positive cells in gut organoids transduced with control (empty bars) or HA-Δ256 FOXO1 adenovirus (black bars). (d,e) Immunohistochemistry with insulin (green), C-peptide (red) and CGA (magenta). (f) Magnification of a typical flask-shaped insulin-positive cell from panele. (g,h) Co-immunohistochemistry with insulin (green), HA (to detect HA-Δ256 Foxo1 adenovirus) (red) and CGA (magenta). (i,j) Co-immunohistochemistry with insulin (green) and FOXO1 (red) or (k,l) insulin (green), α-SMA (red) and CDX2 (magenta). Insets inh,jandlshow magnifications of individual cells. DAPI (blue) was used throughout to visualize DNA. Scale bar, 50 μm ina–e; 10 μm inf(n=3–6 for qPCR and 3 for histology) (*P<0.05 byt-test). We present quantitative data as means±s.e.m. Figure 5: Insulin-positive cells in 184-day-old human gut organoids. ( a , b ) Quantitative PCR (qPCR) analysis of different markers in gut organoids transduced with control (empty bars) or HA-Δ256 FOXO1 adenovirus (black bars). ( c ) Quantification of insulin- and GLP1-positive cells in gut organoids transduced with control (empty bars) or HA-Δ256 FOXO1 adenovirus (black bars). ( d , e ) Immunohistochemistry with insulin (green), C-peptide (red) and CGA (magenta). ( f ) Magnification of a typical flask-shaped insulin-positive cell from panel e . ( g , h ) Co-immunohistochemistry with insulin (green), HA (to detect HA-Δ256 Foxo1 adenovirus) (red) and CGA (magenta). ( i , j ) Co-immunohistochemistry with insulin (green) and FOXO1 (red) or ( k , l ) insulin (green), α-SMA (red) and CDX2 (magenta). Insets in h , j and l show magnifications of individual cells. DAPI (blue) was used throughout to visualize DNA. Scale bar, 50 μm in a – e ; 10 μm in f ( n =3–6 for qPCR and 3 for histology) (* P <0.05 by t -test). We present quantitative data as means±s.e.m. Full size image To provide independent evidence that FOXO1 inhibition increased the generation of insulin-positive cells, we studied 36-day-old organoid cultures. At that stage, insulin-immunoreactive cells were absent in untransduced organoids and INSULIN transcripts were exceedingly low ( Fig. 3u ; Supplementary Table 3 ). In contrast, following transduction with HA-Δ256, we detected insulin-positive cells, albeit at lower frequency than in 184-day-old organoids ( Fig. 6a ). In addition, we used lentivirus encoding FOXO1 small hairpin RNA (shRNA) as an alternative approach to inhibit FOXO1 function. Transduction of 230-day-old organoids with the virus decreased FOXO1 mRNA significantly ( Fig. 6b ), accompanied by the appearance of insulin-immunoreactive cells ( Fig. 6c,d ). Quantitative analyses of the data indicated that insulin-positive cells accounted for 8.5±1.7% of FOXO1-positive cells in organoids transduced with FOXO1 shRNA lentivirus vs 0.8±0.5% in controls ( P <0.05 by t -test). 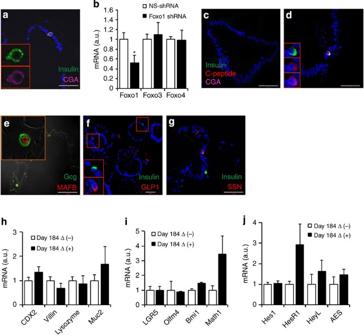Figure 6: Pancreatic lineage marker analysis. (a) Immunohistochemistry with antibodies against insulin (green) and CGA (magenta) in 36-day-old gut organoids transduced with HA-Δ256 FOXO1 adenovirus. (b) Quantitative PCR (qPCR) analysis of 230-day-old gut organoids transduced with control (empty bars) orFOXO1lentiviral shRNA (black bars) (*P<0.05 by ANOVA). (c,d) Immunohistochemistry with anti-insulin (green) and CGA (magenta) antibodies in 230-day-old gut organoids transduced with control orFOXO1shRNA lentivirus. (e) Immunohistochemistry with glucagon (green) and MAFB (red); (f) insulin (green) and GLP1 (red); (g) insulin (green) and somatostatin (red) in 184-day-old gut organoids transduced with HA-Δ256 adenovirus. (h–j) qPCR analysis in 184-day-old gut organoids transduced with control (empty bars) or HA-Δ256 adenovirus (black bars) of transcripts encoding (h) intestinal lineage markers, (i) intestinal stem cell and pan-secretory lineage markers and (j) genes associated with Notch signaling. Figure 6: Pancreatic lineage marker analysis. ( a ) Immunohistochemistry with antibodies against insulin (green) and CGA (magenta) in 36-day-old gut organoids transduced with HA-Δ256 FOXO1 adenovirus. ( b ) Quantitative PCR (qPCR) analysis of 230-day-old gut organoids transduced with control (empty bars) or FOXO1 lentiviral shRNA (black bars) (* P <0.05 by ANOVA). ( c , d ) Immunohistochemistry with anti-insulin (green) and CGA (magenta) antibodies in 230-day-old gut organoids transduced with control or FOXO1 shRNA lentivirus. ( e ) Immunohistochemistry with glucagon (green) and MAFB (red); ( f ) insulin (green) and GLP1 (red); ( g ) insulin (green) and somatostatin (red) in 184-day-old gut organoids transduced with HA-Δ256 adenovirus. ( h – j ) qPCR analysis in 184-day-old gut organoids transduced with control (empty bars) or HA-Δ256 adenovirus (black bars) of transcripts encoding ( h ) intestinal lineage markers, ( i ) intestinal stem cell and pan-secretory lineage markers and ( j ) genes associated with Notch signaling. Full size image In earlier mouse experiments, Foxo1 ablation in gut endocrine progenitors resulted in the appearance of pancreatic glucagon-immunoreactive (α-like) cells, in addition to β-like-cells [6] . Likewise, we found glucagon-/MAFB-positive cells in 184-day-old gut organoids following FOXO1 inhibition, consistent with the generation of pancreatic α-cell-like cells ( Fig. 6e ). The immunoreactivity with MAFB was remarkable, as thus far this α-cell-enriched transcription factor has failed to be induced in endoderm-derived pancreatic endocrine cells [1] . The frequency of glucagon-positive cells in gut organoids transfected with Δ256 was 10% of insulin-positive cells. Notably, we did not see glucagon-positive cells in organoids transduced with control adenovirus at this stage, consistent with an independent effect of FOXO1 inactivation on endocrine cell lineage determination. As insulin-producing cells obtained from embryonic stem or iPS differentiation are often polyhormonal [1] , we investigated whether gut insulin-positive cells are too, but found no evidence that they express other endocrine markers, including GLP1, somatostatin ( Fig. 6f,g ), glucagon and pancreatic polypeptide (PP). FOXO1 loss-of-function did not affect levels of transcripts encoding intestinal stem and pan-secretory markers, including Notch [25] ( Fig. 6h–j ). Marker analysis of insulin-immunoreactive cells Analysis of markers of β-cell differentiation showed that transduction with HA-Δ256 significantly increased transcripts of genes involved in β-cell specification and maturation in 184-day-old gut organoids ( Fig. 7a–c ; Supplementary Table 4 ). It should be noted that NKX2.2 , NKX6.1 and NEUROD transcripts were 10- to 100-fold less abundant than those of other transcription factors ( Supplementary Table 3 ). Immunohistochemistry confirmed that insulin-positive cells were positive for MAFA and UROCORTIN3 ( Fig. 7d–h ). The induction of MAFA—as noted above for that of MAFB–is remarkable, not having been observed in endoderm-derived β-like-cells [1] , [2] , [3] . Insulin-positive cells scored positive for all tested markers of pancreatic β-cells, including PC2, SUR1, PC1/3, glucokinase (GCK) and glucose transporter 2 (GLUT2) ( Fig. 7i–r ) [22] , [26] . 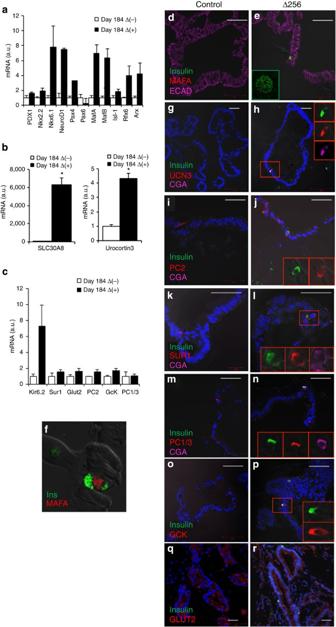Figure 7: Pancreatic marker analysis in 184-day-old gut organoids. (a–c) Quantitative PCR (qPCR) analysis of transcripts of markers associated with β-cell specification and maturation in organoids transduced with control (empty bars) or HA-Δ256 FOXO1 adenovirus (black bars). (d–r) Colocalization of insulin (green) with (d–f) MAFA (the inset in paneleshows green MafA immunoreactivity in human pancreatic islets), (g,h) Urocortin-3, (i,j) PC2, (k,l) SUR1, (m,n) PC1/3, (o,p) glucokinase and (q,r) glucose transporter 2 (all in red). Scale bar, 50 μm ind–r(n=3–6 for qPCR, 3 for histochemistry) (*P<0.05 vs organoids transduced with the control virus byt-test). We present data as means±s.e.m. Figure 7: Pancreatic marker analysis in 184-day-old gut organoids. ( a – c ) Quantitative PCR (qPCR) analysis of transcripts of markers associated with β-cell specification and maturation in organoids transduced with control (empty bars) or HA-Δ256 FOXO1 adenovirus (black bars). ( d – r ) Colocalization of insulin (green) with ( d – f ) MAFA (the inset in panel e shows green MafA immunoreactivity in human pancreatic islets), ( g , h ) Urocortin-3, ( i , j ) PC2, ( k , l ) SUR1, ( m , n ) PC1/3, ( o , p ) glucokinase and ( q , r ) glucose transporter 2 (all in red). Scale bar, 50 μm in d – r ( n =3–6 for qPCR, 3 for histochemistry) (* P <0.05 vs organoids transduced with the control virus by t -test). We present data as means±s.e.m. Full size image Since FOXO1 is predominantly expressed in 5HT cells, we asked whether conversion to insulin-immunoreactive cells following FOXO1 loss-of-function was associated with changes in 5HT expression, using 230-day-old-organoids. Interestingly, we found that transduction with HA-Δ256 adenovirus increased the frequency of CGA-positive cells by approximately twofold, but decreased the number of CGA/5HT-positive cells by ~60% ( P <0.05 by t -test). In contrast, GLP1- and SSN-positive cells were unchanged ( Fig. 4a ). At the cellular level, we observed that the acquisition of insulin immunoreactivity in cells with inactive FOXO1 was associated with loss, or near-complete loss of 5HT immunoreactivity ( Fig. 4b–d ). These data raise the possibility that FOXO1 inhibition activates the insulinogenic program by inhibiting the serotonergic tone of 5HT cells. Converted cells release insulin in response to secretagogoues We investigated whether insulin-positive cells in organoids have the ability to release insulin in a regulated manner. We incubated 200-day-old organoids transduced with HA-Δ256 or control adenovirus with glucose, arginine or KCl. To rule out contamination from insulin present in the medium, we cultured organoids in serum-free medium for 3 days before the experiment, and measured human C-peptide in the supernatant. Under basal conditions, C-peptide was undetectable in organoids. However, it rose to levels between 10 and 20 pmol μg −1 protein in response to 22 mM glucose in control and HA-Δ256 organoids, respectively ( P <0.05 by t -test). Likewise, we observed robust responses to arginine and to the depolarizing agent, KCl. In both instances, HA-Δ256 organoids showed a significantly greater response than controls ( Fig. 8a ). In parallel experiments with collagenase-purified human islets, we estimated that 40 organoids transduced with HA-Δ256 (or 70 untransfected organoids) secrete as much C-peptide as one human islet ( Fig. 8b ). Given the heterogeneity of cellular composition and viability in donor-derived human islets, and in organoids, it is difficult to compare insulin content per cell between the two systems. However, when normalized by protein content, C-peptide secretion in control and HA-Δ256 organoids was 1.0 and 1.6% of human islets, respectively ( Fig. 8a,b ). C-peptide content was significantly higher in gut organoids transduced with HA-Δ256 adenovirus compared with controls ( Fig. 8c ) ( P <0.05 by t -test). 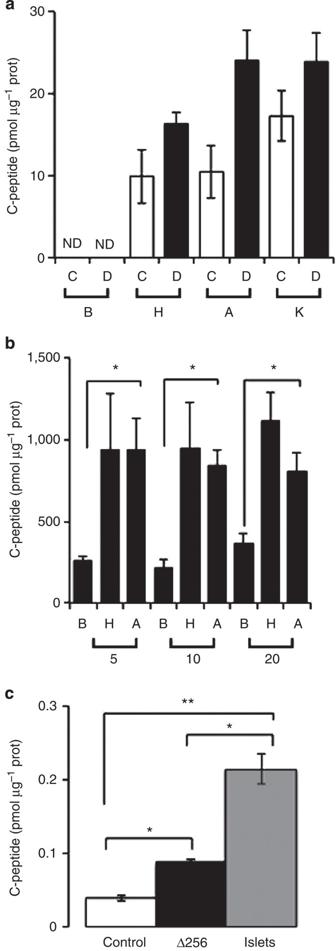Figure 8: Human C-peptide assay using 200-day-old human gut organoids and pancreatic islets. (a) Human C-peptide release from gut organoids normalized by protein levels in organoid lysates. C, control adenovirus; D, HA-Δ256 FOXO1 adenovirus, B, basal glucose (2 mM); H, high glucose (22 mM); A, arginine (10 mM); K, KCl (30 mM); ND, not detected. (b) C-peptide secretion by human islets. Abbreviations are the same as in panela. The numbers below the brackets refer to number of islets used. (c) C-peptide content in gut organoids and human islets *P<0.05 vs organoids transduced with control virus (c) or basal vs glucose- and arginine-stimulated conditions (b) (**P<0.05 vs human islets incbyt-test). We present data as means±s.e.m. (n=3). Figure 8: Human C-peptide assay using 200-day-old human gut organoids and pancreatic islets. ( a ) Human C-peptide release from gut organoids normalized by protein levels in organoid lysates. C, control adenovirus; D, HA-Δ256 FOXO1 adenovirus, B, basal glucose (2 mM); H, high glucose (22 mM); A, arginine (10 mM); K, KCl (30 mM); ND, not detected. ( b ) C-peptide secretion by human islets. Abbreviations are the same as in panel a . The numbers below the brackets refer to number of islets used. ( c ) C-peptide content in gut organoids and human islets * P <0.05 vs organoids transduced with control virus ( c ) or basal vs glucose- and arginine-stimulated conditions ( b ) (** P <0.05 vs human islets in c by t -test). We present data as means±s.e.m. ( n =3). Full size image Transplantation into immunodeficient mice improves the function of endoderm-derived pancreatic β-like-cells [2] , [3] . We tested the effect of transplantation on 200-day-old gut organoids. Owing to their bulkier and anatomically more fragile structure than β-like-cell clusters, we could not safely transplant a sufficient number to detect circulating C-peptide, based on the calculations described above. Nonetheless, we were able to maintain the grafts for 3 weeks, at the end of which they retained an epithelial structure and demonstrated all intestinal lineages, including insulin-positive cells ( Supplementary Fig. 1 ). The number and proportion of β-like-cells was similar to pre-transplantation organoids, indicating that no significant proliferation had occurred in vivo . The present studies provide critical proof-of-principle that gut-targeted FOXO1 inhibition can be used in human iPS-derived gut organoids to increase the efficiency of generating surrogate glucose-responsive, insulin-producing cells. We do not know whether the process of generating insulin-positive cells is a special consequence of the gut organoid system, or can occur in vivo . Nonetheless, it is intriguing that FOXO1 immunoreactivity in the human gut is restricted to endocrine progenitor and serotonin-producing cells, the latter of which are arguably the closest endocrine cell type to an insulin-producing pancreatic β-cell [19] , [27] . There are obvious differences between the various segments of the gut and the organoid system, as exemplified by the spontaneous appearance of insulin-immunoreactive cells in gutoids that were >200-day-old. It is possible that the differentiation conditions employed to generate organoids, with high levels of Wnt signalling [12] , are conducive to the generation of a pancreatic-like endocrine lineage that is not present in vivo. The feasibility of generating insulin-producing cells in the gut has recently received independent confirmation through a related approach, based on combined gain-of-function of three transcription factors, Neurogenin3, MafA and Pdx1 [28] . We do not know whether the two approaches thus far described—FoxO1 loss-of-function and Neurogenin3/MafA/Pdx1 gain-of-function—act through similar mechanisms or even in the same cell type. Interestingly though it has been shown that FoxO1 can inhibit Notch signalling [25] , [29] , which is required for Neurogenin3 activation in the endocrine pancreas, and can directly inhibit Pdx1 in terminally differentiated β-cells [30] . Thus, inhibiting FoxO1 may result in endogenous activation of these genes, as indeed we showed in our original publication [6] . Regardless of whether there is a unifying mechanism behind these observations, the findings indicate that there are multiple ways in which the conversion of gut cells into insulin-producing cells could be achieved. Insulin-immunoreactive cells generated by FOXO1 inhibition display several attractive features: they express markers of terminally differentiated β-cells, such as MAFA, that have proved thus far resistant to induction in endoderm-derived β-like-cells [1] ; they secrete insulin in a strictly stimulus-dependent manner and survive following in vivo transplantation. To augment the efficiency of the conversion process, it will be important in future studies to define its mechanistic relationship to the cell type in which it takes place and to the intracellular pathways involved in it. At this time, we favour a model in which FOXO1 inhibition directly converts 5HT cells into insulin-producing cells by a mechanism that may involve inhibition of 5HT levels and serotonergic tone. But we cannot rule out the possibility that the target cell of FOXO1 inhibition is the NEUROG3 endocrine progenitor cell. This latter possibility is consistent with our mouse studies, in which the appearance of insulin-producing cells occurred following Foxo1 knockout in Neurog3-positive endocrine precursors [6] , and with the observation that in human gutoids, FOXO1 inhibition is associated with an expansion of the CGA-positive cell pool. The latter may allow for the expansion of a rare cell type with the potential to give rise to β-like-cells. Finally, the presence of glucagon-producing cells in organoids following FOXO1 inhibition is also consistent with the generalized de-repression of a pancreatic progenitor-type cell. The approach described here could be used to efficiently generate large quantities of insulin-producing cells for transplantation. However, the goal of our efforts remains to inhibit FOXO1 in vivo , to direct the generation of insulin-producing cells. Such cells would have the advantage of rapid turnover that might allow them to outlast immune attack in type 1 diabetes, and establish a reservoir of self-renewing progenitors that would replenish shed cells. In this regard, optimization of methods for FOXO1 inhibition, including chemical inhibitors [31] , could increase the efficiency of the process. The restriction of FOXO1 expression to serotonin-producing cells in the human gut suggests that FOXO1 manipulation should not affect gut stem cells or other lineages, limiting the potential liabilities of this approach. Hurdles remain, but the present data support the case for further studies in humans. Intestinal samples We obtained specimens of duodenum, jejunum, ileum and colon from patients undergoing intestinal resection procedures or from pancreatic organ donors. We obtained informed consent from individuals or relatives who donated tissue for this study. We processed samples immediately for paraffin embedding by formalin fixation or for frozen section preparation, as described below. The Columbia University Institutional Review Board has approved all procedures. We had ethical approval to carry out this study from the Columbia University Institutional Review Board. Immunohistochemistry We isolated gut organoids from Matrigel, rinsed them in phosphate-buffered saline and fixed them in 4% phosphate-buffered paraformaldehyde for 15 min at room temperature. We fixed human gut specimens in the same buffer overnight. After fixation, we incubated organoids or gut specimens in 30% phosphate-buffered sucrose overnight at 4 °C and embedded them into Cryomold (Sakura Finetek) for subsequent frozen-block preparation. We cut 6-μm-thick sections from frozen blocks, and incubated them with HistoVT One, using Blocking One (both from Nacalai USA) to block nonspecific binding [8] . We incubated sections with primary antibodies for 12 h at 4 °C, followed by incubation with secondary antibodies for 30 min at room temperature. We report catalogue numbers and dilutions used for each antibody in Supplementary Table 1 . We used Alexa-conjugated donkey and goat secondary antibodies (Molecular Probes). After the final wash, we viewed cells using a confocal microscopy (Zeiss LSM 710). We counterstained DNA with 4′,6-diamidino-2-phenylindole (Cell Signaling). For immunostaining of the human gut, we surveyed 100 sets of villi and crypts that could be viewed longitudinally and counted the number and position of enteroendocrine and FOXO1-positive cells. In three independent experiments in the human duodenum, we found 2.8±0.3 CGA-positive, and 2.1±0.4 FOXO1-positive cells per set of villi and crypts. For immunohistochemistry of 200-day-old gut organoids transduced with control and Δ256-HA adenovirus, we pooled at least five organoids, containing on average 5,087±328 and 4,222±851 nuclei, 346±35 and 615±225 CGA-positive cells in one section, respectively ( n =3). For immunohistochemistry of 230-day-old organoids transduced with shRNA lentivirus, we scored at least five organoids for each virus. Each organoid contained an average of 4,546±556 and 4,099±646 nuclei in experiments with the control and FOXO1 shRNA ( n =3). We detected 224±32 and 193±36 FOXO1-positive cells, and 2.0±1.0 and 16.0±3.1 insulin-positive cells in each experiment, respectively. Cell culture We generated human iPS cells from fibroblast of three healthy control subjects as previously described [3] , [4] . Briefly, we obtained upper arm skin biopsies from healthy subject using local anaesthesia. We processed the biopsies as described and placed them culture medium containing DMEM, fetal bovine serum, GlutMAX and penicillin/streptomycin (all from Invitrogen) for 4 weeks [3] . We used the CytoTune-iPS Sendai Reprogramming Kit (Invitrogen) to convert primary fibroblasts into pluripotent stem cells using 50,000 cells per well in six-well dishes Cells were grown in human embryonic stem medium [3] . The Columbia University Institutional Review Board has approved all procedures. We cultured iPS cells in MTeSR (Stemgent) on Matrigel (BD Biosciences)-coated plates and passaged them according to the manufacturer’s instructions. Generation of gut organoids We differentiated human iPS cells into gut organoids as described [23] with some modifications. We used STEMdiff Definitive Endoderm Kit (Stemcell Technologies) instead of Activin A for differentiation towards definitive endoderm. We passaged gut organoids every 2–3 weeks until 360 days and assessed the morphology periodically using immunohistochemistry. We prepared organoids from three different iPS cell lines and performed all experiments using at least three independent biological replicates. In each biological replicate we used at least five organoids for immunohistochemistry and at least three organoids for quantitative reverse transcriptase-PCR (RT-PCR). Adenovirus and lentivirus transduction The recombinant adenoviral vector Ad-CMV-FOXO1-Δ256 expressing a mutant version of FOXO1 containing its amino domain (corresponding to amino-acid residues 1–256) has been described [24] . We prepared adenoviruses by CsCl density centrifugation to a titre of 2.5 × 10 12 viral particles ml −1 (1.6 × 10 11 plaque-forming units ml −1 ) for Ad-CMV-FOXO1-Δ256 and 2.4 × 10 12 vp ml −1 (1.9 × 10 11 p.f.u. ml −1 ) for the Gfp control. Gut organoids were mechanically dissociated from Matrigel, cut in half and incubated in DMEM/F12 containing 10 μM ROCK inhibitor (Y27632) with 1 μl of adenovirus solution for 3 h at 37 °C in a 5% CO 2 incubator and then washed with phosphate-buffered saline three times. After transduction, mini-guts were embedded into fresh Matrigel again and incubated with intestinal growth medium [23] . For lentiviral experiments, we purchased human GIPZ lentiviral FOXO1 shRNA plasmids (Clone ID; V3LHS_405827, 638215, 638212 and 638211, Thermo Scientific) and transfected them in 293 FT cells (Invitrogen) with packaging mix plasmids (Thermo Scientific) using Lipofectamine 2000 (Invitrogen). Plasmids were diluted by Opti-MEM, and Lipofectamine 2000 was added and incubated at room temperature for 20 min. After incubation, the mixture was added to 293 FT cells. We collected viral supernatants 48 and 72 h after transfection and centrifuged them at 6,000 r.p.m. × 2 h to concentrate viral supernatants. Organoid transplantation We transplanted 200-day-old gut organoids transduced with control or HA-Δ256 FOXO1 adenovirus (10 organoids in each group, n =3) under the skin of immunodeficient NOD.Cg- Prkdcscid Il2rgtm1Wjl /SzJ mice (005557; The Jackson Laboratory), using biocompatible ‘Gelfoam’ Dental sponges (size 4) to preserve the anatomy. Three weeks after transplantation, we recovered organoids and performed immunostaining as described above. RNA isolation and RT-PCR We used standard methods of RNA extraction and qRT-PCR (Invitrogen) [6] . Primer sequences are listed in Supplementary Table 2 . C-peptide assay We incubated 200-day-old organoids in serum-free medium for 3 days before the experiment. For each determination, we incubated 10 organoids in 1 ml of Krebs-Ringer buffer containing 10 mM HEPES, 1.19 mM MgSO 4 , 119 mM NaCl, 4.74 mM KCl, 1.19 mM KH 2 PO 4 , 2.54 mM CaCl 2 -2H 2 O, 25 mM NaHCO 3 and 1% bovine serum albumin) and 2.0 mM glucose, at 37 °C for 30 min and replaced the medium and continued the incubation for 30 min. We collected this medium for basal determination. Subsequently, we added 1 ml of Krebs-Ringer buffer containing 22 mM glucose, or 10 mM arginine, or 30 mM KCl and incubated organoids at 37 °C for 30 min, after which medium was collected. At the end of final incubation, organoids were lysed by buffer containing 2% SDS, 50 mM Tris–HCl, 5 mM EDTA and protease/phosphatase inhibitors (Thermo Scientific), sonicated the extract and clarified it by centrifugation. C-peptide secretion and intracellular content of organoids were measured using an ultrasensitive human C-peptide ELISA kit (Mercodia) and protein in lysate was measured using Pierce BCA Protein Assay Kit (Thermo Scientific). We normalized C-peptide release by protein levels in lysates of gut organoids (pmol μg −1 protein). Statistical analysis We used paired or unpaired t -test to determine statistical significance between two groups and one-way analysis of variance for group comparison, with post hoc Bonferroni correction, as appropriate. We used the customary threshold of P <0.05 to declare a statistically significant difference. How to cite this article: Bouchi, R. et al . FOXO1 inhibition yields functional insulin-producing cells in human gut organoid cultures. Nat. Commun. 5:4242 doi: 10.1038/ncomms5242 (2014).